Catalyst-TiO(OH)2could drastically reduce the energy consumption of CO2capture Implementing Paris Climate Accord is inhibited by the high energy consumption of the state-of-the-art CO 2 capture technologies due to the notoriously slow kinetics in CO 2 desorption step of CO 2 capture. To address the challenge, here we report that nanostructured TiO(OH) 2 as a catalyst is capable of drastically increasing the rates of CO 2 desorption from spent monoethanolamine (MEA) by over 4500%. This discovery makes CO 2 capture successful at much lower temperatures, which not only dramatically reduces energy consumption but also amine losses and prevents emission of carcinogenic amine-decomposition byproducts. The catalytic effect of TiO(OH) 2 is observed with Raman characterization. The stabilities of the catalyst and MEA are confirmed with 50 cyclic CO 2 sorption and sorption. A possible mechanism is proposed for the TiO(OH) 2 -catalyzed CO 2 capture. TiO(OH) 2 could be a key to the future success of Paris Climat e Accord. Carbon-based fuels have sustained the world for many centuries. However, their uses have resulted in large amounts of CO 2 emission, a likely cause of the increasingly noticeable climate changes [1] , [2] , [3] , [4] . Thus, CO 2 emission control is imperative by the Paris Climate Accord [5] , [6] . Chemisorption is the most selective and thus promising technology for capturing CO 2 emitted from fossil flue gas due to its simplicity and unique flexibility in dealing with wide concentrations and volumes of CO 2 -containing gases [7] , [8] , [9] . However, its shortcomings are also obvious, including slow sorption and desorption rates. The desorption kinetics is much more important because the CO 2 desorption step typically is much slower and more energy-intensive than the sorption step in the overall CO 2 capture processes. The CO 2 desorption step in conventional CO 2 capture technologies has to be operated at higher temperatures for achieving higher reaction kinetics, typically above 100 °C, which makes this step very expensive, primarily due to the high specific and latent heat capacities of water [10] . How can the absorbed CO 2 be desorbed quickly at temperatures lower than 100 °C—the critical temperature for lowering energy consumption? If the use of catalyst can drastically enhance desorption rates, and thus allow for reducing the CO 2 desorption temperatures, such low desorption temperatures would allow not only for reducing the energy consumption but also utilizing the existing flue-gas waste heat or solar-heated-water, which could completely eliminate the extra energy sources otherwise needed for conventional above 100 °C-desorption based CO 2 capture technologies. A few studies have shown that inorganic materials could be used as catalysts for CO 2 capture. Our group have showed that FeOOH and TiO(OH) 2 could be used as catalytic supports to reduce the activation energy of the NaHCO 3 decomposition reaction and then enhance the decomposition rate [11] , [12] . Idem et al. reported that H-ZSM and γ-Al 2 O 3 could be used to accelerate the amine based solvent regeneration and thus reducing the heat duty for amine regeneration [13] , [14] . Bhatti et al. [15] recently reported an inspiring finding that transition metal oxides could affect spent monoethanolamine (MEA) regeneration. Two of those materials, MoO 3 and V 2 O 5 , were found to improve desorption rates substantially because, in fact, they react and dissolve in the CO 2 -rich MEA solvent. For this reason, they cannot act as a classic, reusable catalyst. The other oxides investigated in that work, including TiO 2 , had only marginal effects. In this work, we find a fundamentally different catalyst in structure—TiO(OH) 2 that can radically change the pathway and thus lower the energy of CO 2 capture. TiO(OH) 2 turns out to be not only very effective in accelerating CO 2 desorption—the key step in CO 2 capture, but also quite stable, and thus a cost-effective CO 2 capture catalyst. A proton transfer based catalytic CO 2 capture mechanism is proposed. Also, the catalysis function of TiO(OH) 2 is supported with both CO 2 desorption experiments and characterization results. Catalytic effect of TiO(OH) 2 on CO 2 absorption and desorption The catalytic effect of TiO(OH) 2 on CO 2 absorption, sorption for short, and desorption using MEA solution as an example is examined in this work with a setup shown in Supplementary Fig. 1 using synthetic flue gas mixture with 10 vol% CO 2 , 10 vol% O 2 , and 80 vol% N 2 . An optimal dosage (Supplementary Fig. 2 ) of 2 wt% TiO(OH) 2 is used for all the tests. 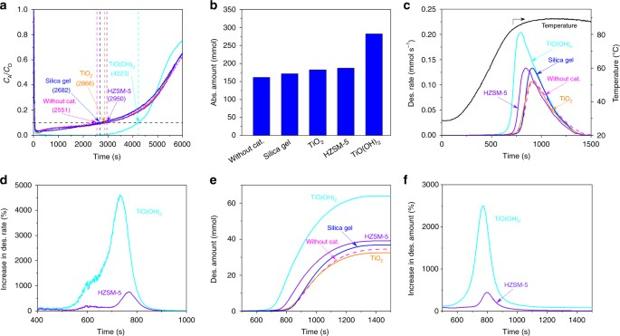Fig. 1 Effect of TiO(OH)2catalyst on CO2absorption (abs.) and desorption (des.).aUncatalyzed and catalyzed CO2absorption profiles of 20 wt% MEA solution.bThe quantities of the CO2sorbed within the effective absorption time (>90% CO2capture).cThe rates of CO2desorption from spent 20 wt% MEA sorbent without and with uses of catalyst (cat.).dThe percentage increases in CO2desorption rate due to the use of TiO(OH)2.eEffects of TiO(OH)2on the quantities of desorbed CO2.fThe percentage increases in CO2desorption amount due to the use of TiO(OH)2. Absorption conditions—total mass of solution: 200 g; MEA concentration in the solution: 20 wt%; total flow rate of gas: 1000 mL/min; composition of gas: 10 vol% CO2, 10 vol% O2, and 80 vol% N2; temperature: 25 °C; absorption time: 6000 s. Desorption conditions—Total mass of solution: 200 g; MEA concentration in the solution: 20 wt%; temperature: 88 °C; time: 2400 s Figure 1a presents CO 2 breakthrough curves for a 20 wt% MEA with and without TiO(OH) 2 , HZSM-5, silica gel, and TiO 2 , all at 2 wt%. Silica gel with similar particle size and porosity to TiO(OH) 2 barely changes the CO 2 sorption breakthrough profile. Qualitatively consistent with the Bhatti et al. work [15] , TiO 2 also barely changes the CO 2 sorption breakthrough curve. Also, recently reported H-ZSM5 [13] , [14] does not change CO 2 breakthrough curve much. However, TiO(OH) 2 significantly increases the effective sorption period in which capturing 90% CO 2 in flue gas is realized as targeted by U.S. Department of Energy (DOE) [16] . The sorbent with longer effective period means that it has higher sorption efficiency and faster CO 2 sorption. The effective sorption time without use of any catalyst and with the use of silica gel, TiO 2 , and HZSM-5 are only 2551, 2682, 2866, and 2950 s, respectively, ~12–16 % increase. While, the period due to use of TiO(OH) 2 jumps to 4223 s, an increase by ~66% in comparison with that without catalyst. Accordingly, the quantities of the CO 2 absorbed without and with uses of TiO(OH) 2 within the corresponding effective sorption times are 162 and 283 mmol, respectively, as presented in Fig. 1b . This represents a 75% improvement. Fig. 1 Effect of TiO(OH) 2 catalyst on CO 2 absorption (abs.) and desorption (des.). a Uncatalyzed and catalyzed CO 2 absorption profiles of 20 wt% MEA solution. b The quantities of the CO 2 sorbed within the effective absorption time (>90% CO 2 capture). c The rates of CO 2 desorption from spent 20 wt% MEA sorbent without and with uses of catalyst (cat.). d The percentage increases in CO 2 desorption rate due to the use of TiO(OH) 2 . e Effects of TiO(OH) 2 on the quantities of desorbed CO 2 . f The percentage increases in CO 2 desorption amount due to the use of TiO(OH) 2 . Absorption conditions—total mass of solution: 200 g; MEA concentration in the solution: 20 wt%; total flow rate of gas: 1000 mL/min; composition of gas: 10 vol% CO 2 , 10 vol% O 2 , and 80 vol% N 2 ; temperature: 25 °C; absorption time: 6000 s. Desorption conditions—Total mass of solution: 200 g; MEA concentration in the solution: 20 wt%; temperature: 88 °C; time: 2400 s Full size image The catalyst effect of TiO(OH) 2 on CO 2 desorption is evaluated with the spent MEA sorbent resulting from 6000 s of CO 2 sorption (Fig. 1a ). The CO 2 desorption study is conducted by heating the CO 2 spent MEA sorbent to a desired desorption temperature under the given heating profile shown in the right y -axis of Fig. 1c . The left y -axis of Fig. 1c shows the changes of the rates of CO 2 desorption from spent 20 wt% MEA sorbent without and with uses of catalysts with time under the same temperatures. 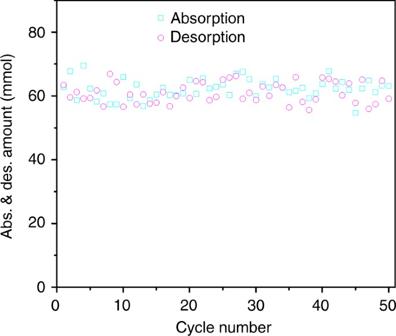Fig. 2 Catalyzed cyclic CO2absorption and desorption. The cyclic tests indicate the stability of TiO(OH)2under the given CO2absorption and desorption conditions. Absorption conditions—total mass of solution: 200 g; MEA concentration in the solution: 20 wt%; total flow rate of gas: 1000 mL/min; composition of gas: 10 vol% CO2, 10 vol% O2, and 80 vol% N2; temperature: 25 °C; absorption time: 6000 and 3000 s for the 1st and 2nd–50th absorption tests, respectively. Desorption conditions—Total mass of solution: 200 g; MEA concentration in the solution: 20 wt%; temperature: 88 °C; time: 2400 s As shown in Fig. 1c , TiO 2 barley changes CO 2 desorption from the spent MEA sorbent. Unlike TiO 2 , the HZSM-5 can slightly improve CO 2 desorption as reported by Idem et al. [13] . Silica gel also can slightly improve CO 2 desorption, however it cannot lower the temperature for maximum CO 2 desorption rate (Supplementary Table 1 ). Compared to the spent MEA without addition of the catalyst, the spent MEA with addition of TiO(OH) 2 could desorb much more CO 2 at the same low temperature range, and have a higher desorption rate at low temperatures. The highest desorption rate of spent MEA with the presence of TiO(OH) 2 reaches 0.204 mmol s −1 at as early as 792 s (Supplementary Table 1 ), while the desorption rates of spent MEAs without the use of TiO(OH) 2 and with the use of HZSM-5 are only 0.0162 mmol s −1 and 0.101 mmol s −1 , respectively, at the same time point. The percentage increases in CO 2 desorption rate due to the use of TiO(OH) 2 and HZSM-5 catalysts as a function of time are presented in Fig. 1d . Remarkably, the increase in the rate of TiO(OH) 2 catalyzed CO 2 desorption can be as high as 4500%, while the highest increase in the rate of HZSM-5 catalyzed CO 2 desorption is only 750%. Therefore, TiO(OH) 2 can significantly catalyze CO 2 desorption, lower CO 2 desorption temperatures required for conventional CO 2 capture technologies, make CO 2 desorption occur at lower than 100 °C operable or practical, and significantly reduce the energy consumption of CO 2 capture. The further extended practical implication of the high CO 2 desorption rate could be its capability in reducing the dimension of amine scrubbing stripper for a given CO 2 capture task. Figure 1e shows the effects of TiO(OH) 2 on the quantities of desorbed CO 2 within the same-time-length cycle of CO 2 sorption and desorption. The drastic enhancement in CO 2 desorption kinetics is illustrated in Fig. 1e with an increase in the total quantity CO 2 desorbed in the same time interval. Only 34.5 mmol CO 2 is desorbed from the spent MEA solution when the catalyst was not used, and the increase of the amount of CO 2 desorbed is ~0% when TiO 2 is used. Silica gel shows a CO 2 desorption amount of 36.9 mmol, a ~7.0% increase. The HZSM-5 slightly improves CO 2 desorption amount to 39.2 mmol, only 14% increase. Extraordinarily, the presence of TiO(OH) 2 leads to a desorption of 64.1 mmol CO 2 , about 86% increase. 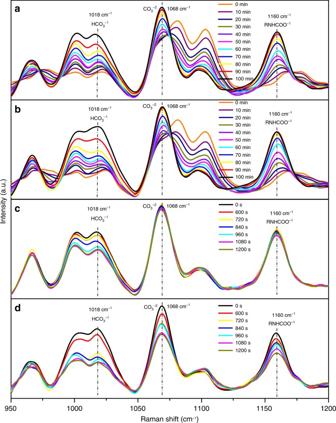Fig. 3 Raman spectra of solutions at different times. The indicated times are the periods when samples were taken during absorption and desorption tests for Raman spectrum analysis. The peak intensities are proportional to the concentration of species in solution.aCO2absorption without TiO(OH)2,bCO2absorption with TiO(OH)2,cCO2desorption without TiO(OH)2,dCO2desorption with TiO(OH)2. Absorption conditions—total mass of solution: 200 g; MEA concentration in the solution: 20 wt%; total flow rate of gas: 1000 mL/min; composition of gas: 10 vol% CO2, 10 vol% O2, and 80 vol% N2; temperature: 25 °C; absorption time: 6000 s. Desorption conditions–total mass of solution: 200 g; MEA concentration in the solution: 20 wt%; temperature: 88 °C; time: 2400 s 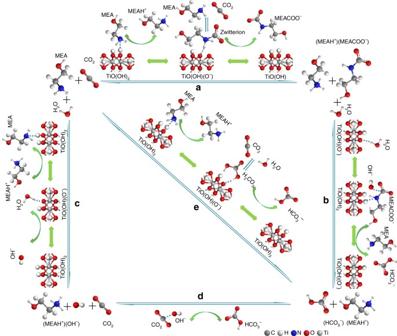Fig. 4 Proposed catalytic mechanism. Three possible pathways for TiO(OH)2to accelerate CO2absorption and desorption with MEA being a sorbent are presented. The hydroxyl group of TiO(OH)2accelerates both protonation and deprotonation reactions and thus CO2capture through reversible sorption and desorption via the special Lewis structure or the dual weak alkalinity and acidity of TiO(OH)2 Although TiO(OH) 2 and HZSM-5 have similar surface areas (Supplementary Table 3 ), the improvement in the quantity of CO 2 desorption resulting from the use of TiO(OH) 2 is 430% higher than that with HZSM-5. It should be mentioned that the difference in CO 2 desorption amounts within a CO 2 sorption-desorption cycle should be much larger than 86% if CO 2 sorption is stopped when CO 2 sorption efficiency falls below DOE-target, 90%. Percentage increase in CO 2 desorption amount due to the use of TiO(OH) 2 and HZSM-5 are provided in Fig. 1f . In comparison with the CO 2 desorption of the uncatalyzed spent MEA, the cumulatively desorbed CO 2 quantity of the catalyzed spent MEA with TiO(OH) 2 is found to be 2500% higher than that of the uncatalyzed spent MEA at 771 s. To avoid the impact of initial CO 2 loading difference on CO 2 desorption, the uncatalyzed and catalyzed CO 2 desorption studies started with two MEA solvents containing the same amount of CO 2 (~0.520 mol CO 2 mol −1 MEA), which are achieved by absorbing CO 2 for 6000 s without the use of TiO(OH) 2 . The desorption results without and with the use of TiO(OH) 2 are summarized in Supplementary Fig. 3 and Table 1 . Clearly, the presence of TiO(OH) 2 catalyst is the main reason for the significantly accelerated CO 2 desorption, given that the initial CO 2 loadings in both spent MEA solvents are the same. The catalytic desorption profile of the spent MEA solvent shows a peak desorption rate of 0.183 mmol s −1 , 168% of the 0.109 mmol s −1 achieved under uncatalyzed desorption condition. The increase in the CO 2 desorption rate resulting from the use of TiO(OH) 2 still can be as high as 2900% in comparison with that achieved without use of TiO(OH) 2 . Accordingly, the total amount of desorbed CO 2 increases from 34.5 mmol to 53.5 mmol with the use of TiO(OH) 2 (Supplementary Fig. 3C ). Catalyst and sorbent stability The stability of TiO(OH) 2 is assessed with 50 cycles of sorption-desorption tests. As shown in Fig. 2 , no obvious decreases in both CO 2 sorption and desorption with the cyclic tests are observed. After cyclic tests, the spent catalyst is filtered, washed, dried, and then characterized by X-ray diffraction (XRD), thermogravimetric analysis (TGA), scanning electron microscope (SEM), and transmission electron microscope (TEM) (Supplementary Figs. 4 – 6 ). These characterization results prove that chemical structure of the TiO(OH) 2 is stable after 50 cyclic tests. The reason for the appearance of tiny XRD peaks of TiO 2 with the spent TiO(OH) 2 is not clear and need to be further studied. FT-IR result of the spent MEA solution (Supplementary Fig. 7 ) shows that MEA also remains stable during the cyclic tests, which may not be the case when it is exposed to the conventionally high regeneration temperatures. Fig. 2 Catalyzed cyclic CO 2 absorption and desorption. The cyclic tests indicate the stability of TiO(OH) 2 under the given CO 2 absorption and desorption conditions. Absorption conditions—total mass of solution: 200 g; MEA concentration in the solution: 20 wt%; total flow rate of gas: 1000 mL/min; composition of gas: 10 vol% CO 2 , 10 vol% O 2 , and 80 vol% N 2 ; temperature: 25 °C; absorption time: 6000 and 3000 s for the 1st and 2nd–50th absorption tests, respectively. Desorption conditions—Total mass of solution: 200 g; MEA concentration in the solution: 20 wt%; temperature: 88 °C; time: 2400 s Full size image Raman spectroscopy Raman spectroscopy is used to investigate the catalytic effect of TiO(OH) 2 on both CO 2 sorption and desorption. To observe the impact of the catalyst on the sorption step, CO 2 sorption with and without TiO(OH) 2 for different sorption periods is performed. The corresponding Raman spectra of the spent MEA sorbents are measured and presented in Fig. 3a and b. The bonds at 1018 cm −1 , 1068 cm −1 , and 1160 cm −1 are attributed to C–OH stretching of HCO 3 − , symmetric C–O stretching of CO 3 2− , and C–N stretching of RNHCO 2 − , respectively [17] . The peak height of RNHCO 2 − generated under catalytic condition reached its highest point more quickly than that without use of the catalyst. Also, the peak intensity of HCO 3 − at the end of the first 100 min of catalyzed CO 2 sorption is stronger than that obtained without use of catalyst. Both Raman spectra observations clearly demonstrate the great effect of the catalyst on CO 2 sorption. On the other hand, Raman spectra of the uncatalyzed and catalyzed CO 2 desorption tests for different periods (0–1200 s) are conducted and the spectra of the resulting MEA solutions are measured and shown in Fig. 3c and d to evaluate the catalytic enhancement effect of TiO(OH) 2 . As can be seen from Fig. 3c , the peak intensity of HCO 3 − in the uncatalyzed desorption derived MEA solution decreased gradually as CO 2 desorption continues, and that of CO 3 2− and RNHCO 2 − does not change during the first 840 s and then started to decrease at a much slower rate with desorption time. However, when desorption is catalyzed, all peak heights of HCO 3 − , CO 3 2− , and RNHCO 2 − in the spent MEA solutions decrease at higher rates. The peak intensity of HCO 3 − in the TiO(OH) 2 -derived MEA solution becomes much weaker within just 720 s, a clear indication of a significant catalytic enhancement of CO 2 desorption due to TiO(OH) 2 . Fig. 3 Raman spectra of solutions at different times. The indicated times are the periods when samples were taken during absorption and desorption tests for Raman spectrum analysis. The peak intensities are proportional to the concentration of species in solution. a CO 2 absorption without TiO(OH) 2 , b CO 2 absorption with TiO(OH) 2 , c CO 2 desorption without TiO(OH) 2 , d CO 2 desorption with TiO(OH) 2 . Absorption conditions—total mass of solution: 200 g; MEA concentration in the solution: 20 wt%; total flow rate of gas: 1000 mL/min; composition of gas: 10 vol% CO 2 , 10 vol% O 2 , and 80 vol% N 2 ; temperature: 25 °C; absorption time: 6000 s. Desorption conditions–total mass of solution: 200 g; MEA concentration in the solution: 20 wt%; temperature: 88 °C; time: 2400 s Full size image Catalytic mechanism A possible catalytic mechanism for TiO(OH) 2 -catalzyed MEA based CO 2 sorption and desorption is proposed in Fig. 4 . There are three possible pathways for bicarbonate formation during CO 2 sorption and MEA regeneration (CO 2 desorption) (Supplementary Fig. 8 ). In the first pathway, forward and reverse steps a and b include carbamate (MEACO 2 − ) generation via a zwitterion intermediate, and then bicarbonate formation through hydrolysis [18] . In the second pathway, one proceeds with forward and reverse formation of (MEAH + )(OH − ), and then bicarbonate, as shown in c and d steps for CO 2 sorption and desorption, respectively. The last one essentially is the association and disassociation of carbonic acid (e and f steps). Protons transfers are directly associated with MEA based CO 2 absorption and desorption [18] . The hydroxyl group of TiO(OH) 2 with the ability of donating and accepting protons can greatly accelerate proton-involved reactions including protonation and deprotonation (Fig. 4 ). For example, TiO(OH) 2 can catalyze steps a and b by providing protons for MEA and accepting protons from zwitterion, which is beneficial to the formation of MEAH + and MEACO 2 − during CO 2 sorption, while it provides protons for MEACO 2 − decomposition and accepts protons for MEAH + deprotonation, which is favorable to sorbent regeneration or CO 2 desorption. Special attention should be paid to critical role of TiO(OH) 2 in the second and third pathways, in which the difficult direct proton transfer from MEAH + to HCO 3 − is avoided via its proton donation to HCO 3 − and deprotonation from MEAH + . Fig. 4 Proposed catalytic mechanism. Three possible pathways for TiO(OH) 2 to accelerate CO 2 absorption and desorption with MEA being a sorbent are presented. The hydroxyl group of TiO(OH) 2 accelerates both protonation and deprotonation reactions and thus CO 2 capture through reversible sorption and desorption via the special Lewis structure or the dual weak alkalinity and acidity of TiO(OH) 2 Full size image Methyl diethanolamine based sorbent To illustrate that the catalytic enhancement of TiO(OH) 2 is not unique to MEA, we use another common amine solvent methyl diethanolamine (MDEA), as an example, as shown in Supplementary Fig. 9 . Comparing Fig. 1 and Supplementary Fig. 9 suggests that TiO(OH) 2 exhibits even stronger catalytic effect on CO 2 desorption from MDEA. Only 2.12 mmol CO 2 is desorbed from the spent 20 wt% MDEA solution when the catalyst is not used. By contrast, the presence of TiO(OH) 2 leads to a desorption of 8.72 mmol CO 2 , about 311% increase. In summary, TiO(OH) 2 can significantly accelerate the both CO 2 sorption and desorption, and lower temperature and thus energy requirements for CO 2 capture. The alleviation in the capture conditions could lead to fundamental changes of people’s passion for CO 2 emission control and successful fulfillment of Paris Agreement. Preparation of TiO(OH) 2 Titanium isopropoxide was used as the precursor for preparing TiO(OH) 2 in this work. The first step was to add a predetermined amount of titanium isopropoxide into deionized (DI) water with a molar ratio of H 2 O:Ti(O-iC 3 H 7 ) 4 being 1400:1, followed by stirring the resulted mixture for 4 h. The precipitate powder was then filtered, rinsed three times with DI water and ethanol, then dried at 100 °C for ~10 h. Characterization The nitrogen physisorption at 77 K was performed on a Quantachrome Quadrasorb SI to determine the surface areas and pore structure of TiO(OH) 2 . Powder X-ray diffraction (XRD) data were obtained by a Rigaku Smart Lab diffraction system with a Cu Kα radiation operated at 40 kV and 40 mA. Thermogravimetric analyses (TGA) of TiO(OH) 2 were performed on a TA Instruments SDT Q600 with a heating ramp of 10 °C min −1 . Fourier transform infrared (FTIR) spectroscopy spectra were collected on a Thermo Nicolet Magna-IR 760 spectrometer. Raman spectrum studies were conducted by using an Advantage 785 Raman Spectrometer with a 758 nm laser and up to 60 mW radiation power during measurement. The samples of MEA sorbents with different absorption and desorption times were prepared by taking about 1 ml solutions with a syringe at specific time, followed by filtering them with syringe filter to remove catalysts, and then placed them in clear shell vials for Raman measurements. Scanning electron microscopy (SEM) images of TiO(OH) 2 were obtained by using a FEI Quanta FEG 450 field-emission scanning electron microscope. Transmission electron microscopy (TEM) images of TiO(OH) 2 were taken by using a FEI Tecnai G2 F20 S-Twin 200 kV transmission electron microscope. CO 2 capture CO 2 absorption and desorption studies were performed by using a setup schematically drawn in Supplementary Fig. 1 . The reactor was a 500 mL glass reactor equipped with a magnetically coupled stirrer. In each sorption test, 200 g of 20 wt% MEA in water was used. Tests were done with or without catalyst. The concentrations (weight percentages) of catalysts varied from 1 wt% to 3 wt%. CO 2 absorption experiment was done at room temperature (~25 °C) and atmospheric pressure (0.78 bar at Laramie in Wyoming). A total of 20 wt% MEA solution was prepared by mixing ethanolamine with deionized water. Predetermined amounts of 20 wt% MEA and catalyst were added into the reactor with a stirring rate of 600 rpm. The simulated flue gas containing 10 vol% CO 2 , 10 vol% O 2 , and 80 vol% N 2 was prepared by mixing individual gases. Three Parker mass flow controllers (Model 201) were used to accurately control the gas flow rates of CO 2 (99.99%), O 2 (99.999%), and N 2 (99.999%) from the corresponding cylinders. The simulated flue gas with a total flow of 1000 ml min −1 was bubbled into MEA solution via a corrosion-resistant muffler (<100 μm, McMaster-Carr). The CO 2 concentration of the outlet gas of the reactor was measured with an inline gas analyzer (NDIR ZRE, California Analytical Instruments), and the measured concentration-time profile was recorded by a data recording unit. The quantity of CO 2 absorbed into MEA solution was calculated by integrating the recorded CO 2 sorption profiles. Upon the completion of absorption step taking 6000 and 3000 s for fresh and cyclic MEA solutions, respectively, the valve for inlet gas was closed. CO 2 desorption was realized by heating the spent sorbent obtained from CO 2 sorption step to a desired desorption temperature (88 °C) gradually. The desorbed CO 2 went through a check valve and mixed with carrier gas (N 2 ) with a flow rate of 500 mL min −1 . The CO 2 concentration of the gas mixture was measured by an in-line gas analyzer (NDIR ZRE, California Analytical Instruments). CO 2 concentrations in the gas mixture and the corresponding temperatures of the spent MEA solution were recorded in the whole CO 2 desorption process. Desorption test was stopped when the concentration of CO 2 in gas mixture was lower than 0.01%. It should be noted the vaporized MEA during CO 2 desorption operation was condensed and sent back to the reactor by using a condenser (#11 in Supplementary Fig. 1 ) along with a cooling unit (#13 in Supplementary Fig. 1 ). The following cyclic CO 2 sorption started to proceed when the temperature of regenerated MEA solution was cooled to 25 °C. CO 2 absorption and desorption experiments with 20 wt% MDEA were conducted by using the same procedures as described earlier. In total 200 g of 20 wt% MDEA was used in the tests. After 6000 s of absorption, CO 2 desorption was realized by heating the spent MDEA sorbent to a desired temperature with the heating profile used for CO 2 desorption from spent MEA sorbent. Data availability The data that support the findings of this study are available from the corresponding author upon request.